Evidence of naturalWolbachiainfections in field populations ofAnopheles gambiae Wolbachia are maternally transmitted intracellular bacteria that invade insect populations by manipulating their reproduction and immunity and thus limiting the spread of numerous human pathogens. Experimental Wolbachia infections can reduce Plasmodium numbers in Anopheles mosquitoes in the laboratory, however, natural Wolbachia infections in field anophelines have never been reported. Here we show evidence of Wolbachia infections in Anopheles gambiae in Burkina Faso, West Africa. Sequencing of the 16S rRNA gene identified Wolbachia sequences in both female and male germlines across two seasons, and determined that these sequences are vertically transmitted from mother to offspring. Whole-genome sequencing of positive samples suggests that the genetic material identified in An. gambiae belongs to a novel Wolbachia strain, related to but distinct from strains infecting other arthropods. The evidence of Wolbachia infections in natural Anopheles populations promotes further investigations on the possible use of natural Wolbachia – Anopheles associations to limit malaria transmission. Malaria-transmitting Anopheles mosquitoes are the deadliest animals on this planet, causing the death of more than 600,000 people each year and endangering the lives of half of the world’s population [1] . Current insecticide-based control strategies to stop malaria transmission by targeting the mosquito vector are limited by the rapid spread of insecticide resistance [2] . In addition, these interventions target only indoor feeding and resting populations, with the use of insecticide-treated bednets and the application of indoor residual sprays, respectively. For decades, the use of Wolbachia endosymbionts has been proposed as an alternative to chemical strategies because of the ability of these bacteria to rapidly invade insect populations via cytoplasmic incompatibility [3] , and successful Wolbachia invasions in field settings have been demonstrated in the case of the dengue and yellow fever vector Aedes aegypti [4] . Recent proof that Wolbachia infections of Anopheles vectors limit the development of the Plasmodium parasites that cause malaria [5] , [6] , [7] , [8] makes these bacteria a particularly attractive tool for the control of both endo- and exophagic populations of malaria-transmitting anophelines. Long-standing limitations concerning the introduction of Wolbachia into laboratory colonies of Anopheles mosquitoes have been recently overcome [5] ; however, the usefulness of this system for the control of Anopheles populations has been undermined by the apparent absence of natural infections. Indeed, while Wolbachia strains have been detected in many insects [9] , [10] , attempts to identify these bacteria in field Anopheles have failed, promoting the belief that these mosquitoes are not natural hosts for Wolbachia [11] , [12] , [13] . In this study, we report evidence of natural Wolbachia infections in two incipient species of the major malaria vector, Anopheles gambiae . We isolate Wolbachia -specific 16S rRNA sequences from the reproductive organs and carcasses of adult mosquitoes and from larval carcasses in three different villages in Burkina Faso, West Africa. Whole-genome shotgun sequencing of two positive samples reveals a previously uncharacterized Wolbachia strain that is maternally transmitted in laboratory settings. These results open new avenues for exploiting Wolbachia infections for field applications targeting the malaria mosquito. Wolbachia sequences detected in field An. gambiae populations We collected mating couples from natural An. gambiae mating swarms in Burkina Faso, West Africa, to identify the microbial populations of the male and female reproductive tracts. We analysed two reproductively isolated populations of An. gambiae , the M and S molecular forms, which do not interbreed in the field [14] and are now classified as two separate species ( An. coluzzii and An. gambiae , respectively [15] ). For simplicity, in the text and in the tables, we will refer to these two species as M and S forms. Our collections included 81 couples captured in three different villages: two villages in Vallée du Kou (VK5 and VK7), where the M form is prevalent, and one village in Soumousso, primarily populated with S form ( Fig. 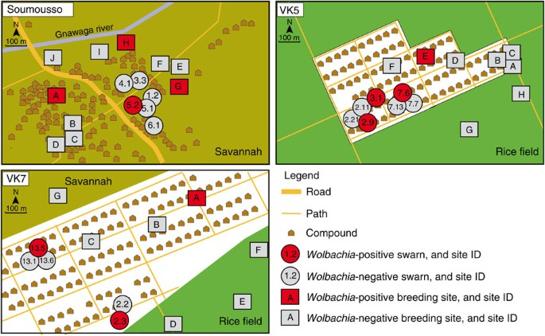Figure 1: Mosquito collection sites and distribution ofWolbachia-infected individuals. The maps describe the three villages (Soumousso, VK5 and VK7) whereAn. gambiaecouples from different mating swarms (indicated by circles) and larvae from different breeding sites (indicated by squares) were collected. Swarm sites and larval breeding grounds are identified by numbers and letters, respectively (seeSupplementary Table 1 and 2). Sites whereWolbachia-positive mosquitoes were found are highlighted in red. Maps were adapted with permission from originals courtesy of A. A. Millogo, IRSS/Centre Muraz, Bobo-Dioulasso, Burkina Faso. 1 , Supplementary Table 1 ). Figure 1: Mosquito collection sites and distribution of Wolbachia -infected individuals. The maps describe the three villages (Soumousso, VK5 and VK7) where An. gambiae couples from different mating swarms (indicated by circles) and larvae from different breeding sites (indicated by squares) were collected. Swarm sites and larval breeding grounds are identified by numbers and letters, respectively (see Supplementary Table 1 and 2 ). Sites where Wolbachia -positive mosquitoes were found are highlighted in red. Maps were adapted with permission from originals courtesy of A. A. Millogo, IRSS/Centre Muraz, Bobo-Dioulasso, Burkina Faso. Full size image An initial high-throughput sequencing of the 16S rRNA gene (variable region V4, average 23,589, s.d. 16,070 assembled reads per sample) amplified from ovaries and testes dissected from 30 mating couples produced a molecular fingerprint of the bacterial population of these reproductive tissues. Surprisingly, this analysis identified one sample, derived from the testes of an S form male collected in Soumousso, infected with Wolbachia . This sample contained 21.8% of reads (5,412 out of 24,800) matching the V4 regions of the Wolbachia 16S rRNA gene, with a percentage identity ranging between 95.3 and 97.6%. This percentage is fully consistent with the overall diversity of known Wolbachia V4 sequences (average identity 95.9%, s.d. 1.75%, median 96.0% as estimated from available sequences, see Methods), while it is incompatible with any other sequenced bacterial 16S gene (closest matches at <89% identity). Phylogenetic analysis rooted the Wolbachia sequences into one of the two main subtrees of the genus, further confirming their taxonomic placement ( Fig. 2 ). 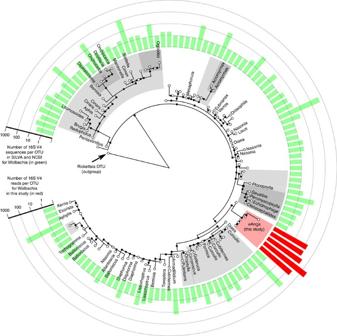Figure 2: Phylogenetic tree forWolbachia 16SrRNA sequences. The tree was built using V416SrRNA fragments fromWolbachiareference sequences available in public repositories (NCBI and SILVA) and from the sequences obtained in this study. The sequences are clustered at 99% identity and the cardinality of each OTU obtained is reported in a logarithmic scale as a bar chart external to the tree (green for reference sequences and red for the new sequences). Shadings highlight subtrees with high bootstrapping support (>90%) and host organisms are reported for those OTUs in which at least one-third of the sequences are consistently associated to the same host. Figure 2: Phylogenetic tree for Wolbachia 16S rRNA sequences. The tree was built using V4 16S rRNA fragments from Wolbachia reference sequences available in public repositories (NCBI and SILVA) and from the sequences obtained in this study. The sequences are clustered at 99% identity and the cardinality of each OTU obtained is reported in a logarithmic scale as a bar chart external to the tree (green for reference sequences and red for the new sequences). Shadings highlight subtrees with high bootstrapping support (>90%) and host organisms are reported for those OTUs in which at least one-third of the sequences are consistently associated to the same host. Full size image The identification of Wolbachia sequences in the testes of an An. gambiae male prompted us to analyse the remaining mosquito specimens collected from the same mating swarms in the three villages. To this aim, a more sensitive PCR-based amplification and sequencing of a 16S rRNA gene segment comprising three variable regions (V6, V7 and V8) was utilized to specifically detect Wolbachia in ovaries and testes dissected from the remaining 51 mating couples, using previously validated primers [16] . The mosquito carcasses were also examined using the same method. Out of the 102 mosquitoes analysed, 11 were positive for Wolbachia 16S rRNA, leading to a frequency of infection of 10.8% similarly distributed between males and females (5 males and 6 females) ( Supplementary Table 1 ). Interestingly, Wolbachia sequences were PCR amplified from either the reproductive tissues or from the carcasses, but never from both, with the exception of one male, where 16S sequences were identified by high-throughput sequencing in the testes and by PCR in the carcass. Although sequences corresponding to these endosymbionts were more prevalent in M mosquitoes, the difference in frequency between the two species was not statistically significant (12.8% in M samples compared with 4.2% in S samples). We also amplified DNA from fourth instar larvae collected from the same three villages (100 specimens from Soumousso, 80 specimens from VK5 and 70 specimens from VK7) using the same primer sets described above. Wolbachia sequences were found in five larval samples (three from Soumousso, one from VK5 and one from VK7), suggesting occurrence of maternal transmission ( Supplementary Table 2 ). Wolbachia sequences group into two different clusters Analysis of the amplified regions determined the presence of at least two distinct clusters of Wolbachia sequences ( Supplementary Fig. 1 ). One cluster was identical to the reference strains w AlbB isolated from A. albopictus [17] , while the second was closely related to several w Pip strains isolated from Culex mosquitoes and Drosophila species [18] . The w AlbB-like cluster was detected only in reproductive tissues (ovaries and testes), while w Pip-like sequences were more widespread and were found in ovaries, carcasses and whole larvae ( Supplementary Fig. 1 ). Although these Wolbachia ribosomal sequences are not host specific, the identification of two distinct clusters suggests the occurrence of independent Wolbachia infections in An. gambiae , as observed in other hosts [19] . We next analysed the distribution of the Wolbachia sequences among the different villages. A larger number of positive individuals were isolated from mating swarms in VK5, where 7 out of the 36 collected mosquitoes showed evidence of infection (19.4%). The other 4 positive samples were found in VK7 (3 samples out of 42, 7.1%) and Soumousso (1 sample out of 24, 4.2%) ( Supplementary Table 1 ). Strikingly, six of the seven positive samples isolated from VK5 had been collected in just two of the seven mating swarms analysed in that village ( Supplementary Table 1 ). If confirmed, such clustering of Wolbachia -positive individuals in specific swarms would suggest that ecological and environmental factors might play a key role in the establishment of Wolbachia infections in the An. gambiae host. The Wolbachia strain belongs to a new phylogenetic group To expand the 16S rRNA-based analysis and better characterize the Wolbachia strain found in An. 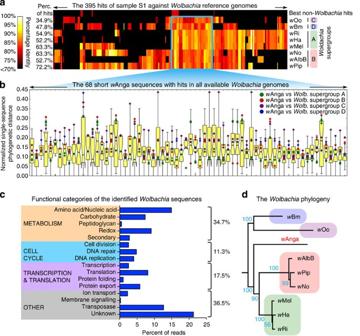Figure 3: Whole-genome shotgun sequencing of aWolbachia-positive sample identifies a newWolbachiastrain inAn. gambiae. Ovaries from aWolbachia-positive female (sample S1) were sequenced using WGS. (a) Percentage (Perc.) identity of 395 short sequences uniquely attributable toWolbachiafrom sample S1 versus eight sequenced strains. TheWolbachiareference strains and the supergroups are indicated with the corresponding percentage of assigned sequences. (b) Distribution of phylogenetic distances between differentWolbachiasupergroups, from phylogenies reconstructed separately on each of the short sequences universally conserved withinWolbachiagenomes (light blue inset ina). (c) Functional classification ofWolbachialoci identified by alignment to read sequences, based on NCBI annotated gene functions. (d)Wolbachiaphylogeny, comprising the newWolbachiastrainwAnga isolated inAn. gambiae, reconstructed from the concatenated sequences ofb. These analyses show thatwAnga is different from all other strains sequenced so far. The same analyses for another PCR-positiveWolbachiasample are available inSupplementary Fig. 3. gambiae , we performed whole-genome shotgun (WGS) metagenomic sequencing of two of the Wolbachia -positive samples from mosquito ovaries ( Supplementary Table 3 ). Sequences corresponding to the An. gambiae genome were screened out, and a pipeline for detecting Wolbachia -specific sequences based on the unique marker approach was applied [20] (see Methods). A total of 571 reads uniquely attributable to Wolbachia were detected ( Fig. 3a,b , Supplementary Fig. 3a,b ) with 86±3.9 and 87.0±4.4% average identity for the two samples analysed, which is in line with the sequence divergence observed for Wolbachia strains in different supergroups ( Supplementary Fig. 2 ). These sequences matched 134 Wolbachia genes belonging to different functional categories ( Fig. 3c , Supplementary Fig. 3c ). The majority of reads (32.2% on average across the two samples) matched genes from metabolic pathways, while a relevant number of reads (13.3%) corresponded to Wolbachia -specific transposases; this is in line with the observation that transposases abundantly populate the genome of Wolbachia strains from many insects including mosquitoes (for example, transposases correspond to 8.32% of all genes annotated in the w Pip genome [18] ). 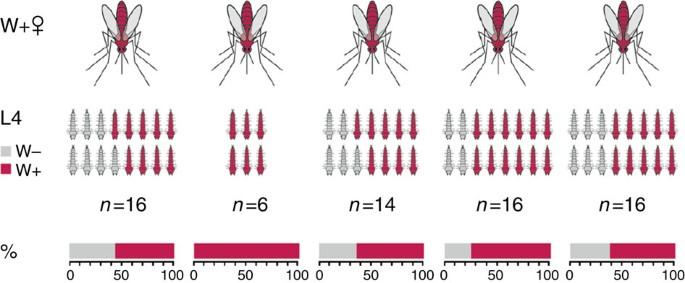Figure 4: Vertical transmission ofWolbachiafrom mother to offspring. A total of 14Wolbachia-positive blood-fedAn. gambiaefemales collected from houses in VK5 were allowed to lay eggs individually. The progeny of the fiveWolbachia-positive females (W+) that laid eggs was screened for the presence ofWolbachiaat the fourth larval developmental stage (L4). Red indicatesWolbachia-positive larvae and adults. The number of larvae screened is shown for each female (n). Alignment of our reads to eight fully or partially sequenced Wolbachia reference genomes ( Supplementary Table 4 ) demonstrated that the strain identified here belongs to a potential Anopheles -specific phylogenetic supergroup, distinct from the arthropod-associated and evolutionarily related supergroups A and B ( Fig. 3d , Supplementary Fig. 3D ). We henceforth call this strain w Anga. Figure 3: Whole-genome shotgun sequencing of a Wolbachia -positive sample identifies a new Wolbachia strain in An. gambiae . Ovaries from a Wolbachia -positive female (sample S1) were sequenced using WGS. ( a ) Percentage (Perc.) identity of 395 short sequences uniquely attributable to Wolbachia from sample S1 versus eight sequenced strains. The Wolbachia reference strains and the supergroups are indicated with the corresponding percentage of assigned sequences. ( b ) Distribution of phylogenetic distances between different Wolbachia supergroups, from phylogenies reconstructed separately on each of the short sequences universally conserved within Wolbachia genomes (light blue inset in a ). ( c ) Functional classification of Wolbachia loci identified by alignment to read sequences, based on NCBI annotated gene functions. ( d ) Wolbachia phylogeny, comprising the new Wolbachia strain w Anga isolated in An. gambiae , reconstructed from the concatenated sequences of b . These analyses show that w Anga is different from all other strains sequenced so far. The same analyses for another PCR-positive Wolbachia sample are available in Supplementary Fig. 3 . Full size image w Anga is maternally transmitted The presence of Wolbachia DNA in the reproductive tissues of female adults prompted the question of whether these bacteria are inherited from mother to offspring, an essential prerequisite for their spread through a population. To obtain irrefutable proof of vertical transmission and estimate its efficiency, semi-gravid females were collected from houses in VK5 two seasons after the initial collections. The same sets of Wolbachia 16S fragments were identified at a frequency of 21% (19 out of 91 females), and the progenies of the 5 Wolbachia -positive females that laid eggs were then analysed for infection. Occurrence of maternal transmission was detected in all progenies, with an average transmission frequency of 68% (ranging from 56 to 100%) ( Fig. 4 ). Taken together, these data confirm the presence of Wolbachia sequences over the course of 2 years and indicate occurrence of vertical transmission from mother to offspring, as normally observed in Wolbachia infections. Figure 4: Vertical transmission of Wolbachia from mother to offspring. A total of 14 Wolbachia -positive blood-fed An. gambiae females collected from houses in VK5 were allowed to lay eggs individually. The progeny of the five Wolbachia -positive females (W+) that laid eggs was screened for the presence of Wolbachia at the fourth larval developmental stage (L4). Red indicates Wolbachia -positive larvae and adults. The number of larvae screened is shown for each female ( n ). Full size image The identification of genomic sequences from a novel Wolbachia strain in two incipient species of An. gambiae over the course of different seasons suggests that anopheline mosquitoes naturally harbour these bacteria, prompting renewed efforts to exploit Wolbachia to block malaria transmission. Past attempts to identify Wolbachia in these mosquitoes may have failed due to possible methodological limitations in the detection systems used, including non-optimal DNA amplification and extraction methods, and size of the sampled mosquito population [11] , [12] , [13] . In addition, the newly identified w Anga strain appears to be highly divergent from Wolbachia strains isolated in other insects. Indeed, our attempts to amplify by PCR two Wolbachia -specific genes commonly used in phylogenetic analyses, the wolbachia surface protein wsp and the fructose-biphosphate aldolase fbpA , were unsuccessful despite numerous attempts (see Supplementary Table 5 for primer sets used), suggesting a low degree of sequence conservation. Interestingly, in some Wolbachia strains infecting C. pipiens , the wsp B gene is disrupted by the insertion of an IS256 transposon [21] , which belongs to the same family of transposons identified in w Anga. Similar transposon insertions into wsp may have occurred in the Wolbachia strain infecting An. gambiae , compromising the amplification of this gene. Although examples of horizontal gene transfer (HGT) between Wolbachia and insect hosts are widespread [22] , [23] , two major observations strongly argue against the possibility of HGT of Wolbachia sequences into the An. gambiae genome: (1) with one exception, evidence of infection was identified in reproductive tissues (ovaries and testes) from nine females and males but not in the carcasses dissected from the same individuals, or vice versa, ruling against a possible transfer into the mosquito chromosomes; (2) the average coverage of Wolbachia in our WGS samples was lower than 0.05 × , which is incompatible with the three orders of magnitude higher coverage of the An. gambiae genome in the same samples (>75 × ). Alternatively, HGT may have occurred into a bacterium or eukaryotic microorganism that infects the Anopheles germline and is maternally inherited from mother to progeny (based on the evidence of vertical transmission of 16S sequences). Regardless of their origin, the Wolbachia sequences identified here may still be sufficient to induce Wolbachia- like reproductive phenotypes, such as bidirectional cytoplasmic incompatibility, that would impact future field deployments of experimental Wolbachia infections [4] . The unexpected discovery in the mosquito germline of maternally inherited Wolbachia organisms will prompt further studies of the ecological, environmental and genetic determinants of susceptibility of Anopheles mosquitoes to Wolbachia infections. It will also spark critical investigation into whether natural Wolbachia–Anopheles associations limit the development of Plasmodium parasites in the mosquito host, thus aiding the design of novel effective bacterial infection strategies to control malaria transmission. Mosquito collections Mosquito samples were initially collected during August–September 2011 in three different sites near Bobo-Dioulasso, Burkina Faso. The village of Soumousso (11°00′N; 4°02′W) is located 55 km North-East of Bobo-Dioulasso. It is characterized by wooded savannah and by temporary breeding sites, more favourable to S form ( An. gambiae ) [14] . The two other collection sites are located in Vallée du Kou, a large rice-growing area situated 30 km North-West of Bobo-Dioulasso. The village of VK5 (11°23′N; 4°24′W) is completely surrounded by rice fields, while VK7 (11°24′N; 04°24′W) is characterized by rice fields to the South and by Savannah to the North. Because of the irrigation system, rice fields form permanent mosquito breeding sites in which the M form ( An. coluzzii ) thrives [14] . Nonetheless, few transient breeding sites could be found in depressions and ponds within the villages. Male and female adult mosquitoes were collected in copula [24] from an average of six mating swarms per collection day. Fourth instar larvae were also collected from temporary and permanent water pools from each site. A schematic representation of the villages and swarm locations is provided in Fig. 1 . In August 2013, blood-fed An. gambiae females were collected inside the houses in VK5 and allowed to individually oviposit in the insectary. DNA extraction and species genotyping Genomic DNA was extracted from dissected reproductive tissues (testes and ovaries) using DNeasy kit (Qiagen), and from carcasses using NucleoSpin 96 Tissue kit (Macherey-Nagel). In 2013, to estimate Wolbachia maternal transmission, DNA was extracted using DNeasy kit (Qiagen) from whole females that were allowed to oviposit, and from their progenies. For M and S genotyping, DNA was extracted from a leg using a fast extraction method. In brief, individual legs were incubated in 40 μl of grinding buffer (10 mM Tris-HCl pH 8.2, 1 mM EDTA, 25 mM NaCl) with 0.2 mg ml −1 proteinase K for 45 min at 37 °C, then 5 min at 95 °C to inactivate the enzyme. DNA extracts (1 μl) were then subjected to PCR amplification targeting the locus S200 × 6.1 using specific primers (FWD: 5′-TCGCCTTAGACCTTGCGTTA-3′; and REV: 5′-CGCTTCAAGAATTCGAGATAC-3′) [25] . M and S genotyping was also used on larvae and adult carcasses. Larval DNA was used to determine the sex using Y-specific primers (F: 5′-CAAAACGACAGCAGTTCC-3′; and R: 5′-TAAACCAAGTCCGTCGCT-3′). 16S rRNA profiling and sequencing The 16S rRNA gene data set consisted of Illumina MiSeq sequences targeting the V4 variable region. Detailed protocols used for 16S amplification and sequencing were previously described [26] . In brief, genomic DNA from testes and ovaries was subjected to 16S rRNA amplifications using primers incorporating the Illumina adapters and a sample barcode sequence, allowing directional sequencing covering the variable region V4 (15F: 5′-GTGCCAGCMGCCGCGGTAA-3′; and 806R: 5′-GGACTACHVGGGTWTCTAAT-3′). PCR mixtures contained 10 μl of diluted template (1:50), 10 μl of HotMasterMix with the HotMaster Taq DNA Polymerase (5 Prime) and 5 μl of primer mix (2 μM of each primer). The cycling conditions consisted of an initial denaturation at 94 °C for 3 min, followed by 30 cycles of denaturation at 94 °C for 45 s, annealing at 50 °C for 60 s, extension at 72 °C for 5 min and a final extension at 72 °C for 10 min. Amplicons were quantified on the Caliper LabChipGX (PerkinElmer, Waltham, MA), pooled in equimolar concentrations, size selected (375–425 bp) on the Pippin Prep (Sage Sciences, Beverly, MA) to reduce nonspecific amplification products from host DNA and a final library size and quantification was done on an Agilent Bioanalyzer 2100 DNA 1000 chips (Agilent Technologies, Santa Clara, CA). Sequencing was performed on the Illumina MiSeq v2 platform, according to the manufacturer’s specifications with addition of 5% PhiX, generating paired-end reads of 175 bp in length in each direction. The overlapping paired-end reads were stitched together (~\n97 bp overlap) and size selected to reduce nonspecific amplification products from host DNA (225–275 bp). High-throughput 16S rRNA screening We first applied the QIIME pipeline version 1.6 (ref. 27 ) to the 16S rRNA data set that detected in the testis sample G23656 (male SMS5.1 in Supplementary Fig. 1 ) a total of 19.9% of reads assigned to Wolbachia . To specifically investigate and validate the prediction about the presence of Wolbachia in the sample, we implemented an additional pipeline. We first integrated all 16S rRNA sequences assigned to Wolbachia included in the SILVA [28] and NCBI repositories; we manually inspected those sequences with a >3% nucleotide divergence from any other Wolbachia 16S , which let us exclude five sequences that were mislabeled with close endosymbionts such as Bartonella , Rickettsia and Francisella . We obtained a set of 2,064 Wolbachia 16S sequences from which the 253-nt-long V4 region was extracted and clustered at 99% identity, generating 115 operational taxonomic units (OTUs) covering the diversity in the Wolbachia genus. The all-versus-all mapping of the 115 OTU sequence representatives provided a lower-bound estimate of the genus’ total diversity (average identity of 95.9%, s.d. 1.75%, median 96.0%). We then performed the mapping of the 24,800 reads of sample G23656 against the full SILVA database, retaining only those sequences with full-length percentage identity of at least 95% with a Wolbachia 16S . The resulting 5,412 reads have a best hit other than Wolbachia at <89% identity, confirming that a fifth of the sample (21.82%) consists of V4 fragments from Wolbachia 16S rRNA. The percentage identity was in the 95.3–97.6% interval, which is fully consistent with the observed diversity in the V4 hypervariable region of the Wolbachia 16S rRNA genes (average 95.9%, s.d. 1.75% as reported above). The V4 sequences from sample G23656 were then clustered into OTUs at 99% identity, discarding those OTUs with <50 sequences. The resulting OTUs were merged with the Wolbachia OTUs from the SILVA and NCBI repository (generated as described above) and aligned with MUSCLE version 3.8.31 (ref. 29 ). A V4 sequence representative of the Rickettsia 16S was added as outgroup. A phylogenetic tree was then built using RAxML version 7.4.2 (ref. 30 ) with the GTRGAMMA model, bootstrapping (1,000 replicates), best maximum likelihood tree inference, and displayed with GraPhlAn ( https://bitbucket.org/nsegata/graphlan ) representing the cardinality of the OTUs as circular barplots. Wolbachia -specific PCR detection and sequencing DNA from testes and ovaries was rehydrated from the 96-well Qiasafe plate (Qiagen) using 30 μl of water. A total of 2 μl of DNA was used for Wolbachia PCR detection using primers specific for Wolbachia 16S rDNA (W-Specf 5′-CATACCTATTCGAAGGGATAG-3′, W-Specr 5′-AGCTTCGAGTGAAACCAATTC-3′) following standard procedures [16] . Positive samples showed a 438-bp band that was purified with QIAquick Gel Extraction kit (Qiagen) and sequenced (Eurofins MWG Operon, Ebersberg, Germany). Sample DNA quality was assessed with PCR using primers for the RpS7 (AGAP010592) An. gambiae gene (FWD 5′-GGCGATCATCATCTACGTGC-3′; and REV 5′-GTAGCTGCTGCAAACTTCGG-3′). Similarly, a total of 2 μl of DNA was used for PCR detection of wsp and fbpA genes following standard procedures (see Supplementary Table 5 for primer sets used). WGS sequencing and analysis pipeline Shotgun metagenomic sequencing was performed on two mosquito samples from infected ovaries using the remainder of the DNA available after Wolbachia- specific PCR detection (1–2 ng). Due to this limiting condition, libraries were prepared with 1 ng DNA according to the Nextera XT protocol (Version Oct 2012). Briefly, the DNA was fragmented in 5 μl of Amplicon Tagment Mix and 10 μl of Tagment DNA buffer (Illumina, San Diego, CA, USA). Tagmentation reactions were completed by incubation for 5 min at 55 °C followed by neutralization with 5 μl of Neutralise Tagment Buffer for 5 min. Tagmented DNA was used as the template in a 50-μl limited-cycle PCR (12 cycles) and processed as described in the Nextera XT protocol. Amplified DNA was purified with AMPure XP beads and then normalized to 2nM. Sequencing was performed on a HiSeq2000 (Illumina, San Diego, CA, USA) employing one full lane per library with 101 bp paired-end reads. Raw WGS results consisting of >400 M 101-nt-long paired-end reads ( Supplementary Table 3 ) were subject to quality control and sliding window trimming with a minimum resulting read length of 80 bp, and to sequencing artefact removal using PRINSEQ version 0.20.3 (ref. 31 ). As expected, An. gambiae DNA was quantitatively dominant in the read pool, and was removed by BowTie2 mapping [32] using the ‘very-sensitive’ preset option against the An. gambiae PEST reference genome ( http://www.vectorbase.org/ ). Supplementary Table S2 reports the number of reads that were retained after each pre-processing step. The resulting read set was mapped against the seven available Wolbachia genomes and the high-quality draft assembly of the Wolbachia strain w AlbB ( Supplementary Table 4 ). To quantify the expected sequence divergence between Wolbachia strains and supergroups, we performed all-versus-all sequence mapping (with BLASTN) with all open reading frames (ORFs), considering as pairwise common ORFs those sequences with >80% identity over 50% of the ORF length ( Supplementary Fig. 2 ). Reads were uniquely attributable to Wolbachia on the basis of the concept of unique marker sequences [20] , performed in four steps. First step: BowTie2 mapping against the eight Wolbachia reference genomes was performed to identify Wolbachia candidate reads. The mapping was performed with enhanced sensitivity (score-min L,-1.0,-1.0 -D 25 -R 5 -N 1 -L 12 -i S,2,0.25) to capture Wolbachia sequence divergence and host specificity as assessed by ORFs’ sequence comparison among available Wolbachia genomes ( Supplementary Fig. 3 ). The matches were also confirmed by BLASTN with word size of length 7. Second step: candidate reads coming from the small and large ribosomal units ( 16S rRNA and 23S rRNA genes) were screened out by sequence mapping against the comprehensive ribosomal sequences in the SILVA database release 111. Third step: the remaining ribosomal-free candidate reads were mapped against the full RefSeq genomic database version 60 to identify any non- Wolbachia -specific hits using BLASTN with word size of length 7. Fourth step: on the basis of the mapping results of steps 1 and 3, the final set of reads from the Wolbachia strain identified in An. gambiae ( w Anga) was compiled selecting all reads showing >80% identity over >95 nt to at least one Wolbachia strain, and no hits longer than 80 nt to other organisms. Reads hitting non- Wolbachia genomes with identities below 80% and at least one Wolbachia genome at >90% were also retained. As control, the same procedure was also applied to the two genera closest to Wolbachia according to the PhyloPhlAn tree of life [33] , namely, Anaplasma (six reference genomes) and Ehrlichia (five reference genomes). No uniquely attributable reads were found in this analysis. w Anga reads mapping to all seven Wolbachia genomes were then retained for phylogenetic analysis. The homologous sequences were extracted and aligned to each w Anga reads with MUSCLE version 3.8.31 (ref. 29 ) and the alignments edited to remove leading and ending gaps. Sequence-specific phylogenetic trees were built using RAxML version 7.4.2 (ref. 30 ) with the GTRGAMMA model, bootstrapping (1,000 replicates) and best maximum likelihood tree inference. Sequence-specific phylogenetic distances were computed inferring the patristic distances within each tree, and reported with box plots in Fig. 3b and Supplementary Fig. 3B . A final phylogenetic tree was also built using RAxML (GTRGAMMA model, 1,000 bootstrapping replicates) on the concatenated alignments ( Fig. 3d , Supplementary Fig. 3D ). Accession codes: Nucleotide sequences of PCR-amplified fragments of Wolbachia 16S rRNA genes have been deposited in the GenBank nucleotide database under accession codes KJ728739 to KJ728755 . Sequence reads for the same 16S-rRNA amplicon sequences have been deposited in the NCBI Sequence Read Archive (SRA) under accession code SRR610826 . Sequence reads for the two whole-genome shotgun sequencing samples have been deposited in the NCBI Sequence Read Archive (SRA) under accession codes SRR1238105 to SRR1238106 . How to cite this article: Baldini, F. et al. Evidence of natural Wolbachia infections in field populations of Anopheles gambiae . Nat. Commun. 5:3985 doi: 10.1038/ncomms4985 (2014).